Carbon arc production of heptagon-containing fullerene[68] A carbon heptagon ring is a key unit responsible for structural defects in sp 2 -hybrized carbon allotropes including fullerenes, carbon nanotubes and graphenes, with consequential influences on their mechanical, electronic and magnetic properties. Previous evidence concerning the existence of heptagons in fullerenes has been obtained only in off-line halogenation experiments through top-down detachment of a C 2 unit from a stable fullerene. Here we report a heptagon-incorporating fullerene C 68 , tentatively named as heptafullerene[68], which is captured as C 68 Cl 6 from a carbon arc plasma in situ . The occurrence of heptagons in fullerenes is rationalized by heptagon-related strain relief and temperature-dependent stability. 13 C-labelled experiments and mass/energy conservation equation simulations show that heptafullerene[68] grows together with other fullerenes in a bottom-up fashion in the arc zone. This work extends fullerene research into numerous topologically possible, heptagon-incorporating isomers and provides clues to an understanding of the heptagon-involved growth mechanism and heptagon-dependent properties of fullerenes. Cage-closed all-carbon structures, including fullerenes and carbon nanotubes, are typically composed of hexagon and pentagon carbon rings [1] , [2] . Experimentally, however, heptagon rings are also incorporated into carbon frameworks making the experimentally available carbon allotropes (for example, fullerenes and carbon nanotubes, as well as graphenes) defective species [3] , [4] , [5] , [6] , [7] , [8] , [9] , [10] . Although unambiguous identification of heptagons in the family of all-carbon allotropes remains an open question, numerous theoretic studies have focused on the heptagon-involved defect because of its key responsibility for changing geometric structures and properties of the experimentally available carbon allotropes [11] , [12] , [13] , [14] , [15] , [16] , [17] , [18] , [19] . The possible existence of heptagons in carbon nanotubes was first proposed by Iijima [3] in 1992. A heptagon-incorporating fullerene, named a heptafullerene in this work, was originally proposed by Taylor [20] . Heptafullerene[72], which has been predicted by Akasaka and Nagase [21] from 431,240 isomeric possibilities, is more stable than the Isolated Pentagon Rule [22] satisfying isomer in form of endofullerene Ca@C 72 . A bare heptafullerene[62] with C s -symmetry [23] , as well as the exohedral heptagon-containing C 68 X 4 (X=H, F, Cl) [24] , has been calculated to be more stable than all the classical non-heptagon isomers. Very recently, a number of smaller heptafullerenes (C 46 –C 58 ) have also been suggested to be viable [18] , [25] , [26] . However, experimental confirmation of the existence of heptagons in the family of fullerenes is still a challenge for chemists and physicists. It is possible chemically to manipulate a few of the carbons on a fullerene surface to modify the carbon cages into heptafullerene derivatives, such as C 58 F 18 (ref. 27 ) and C 84 Cl 32 (ref. 28 ). Such work has provided a breakthrough in the synthesis of heptafullerene derivatives by a top-down chemical method. Clearly, such synthetically produced halides of heptafullerenes (C 58 and C 84 ) are not species directly retrieved from an in situ carbon-clustering process. Thus, these species do not establish the finite existence of unmodified heptafullerenes. Here we perform an experiment, using graphite arc-discharge, which is well known for bottom-up growth of the whole family of sp 2 -hybrided carbon allotropes [2] , [29] , [30] , to capture a heptafullerene[68] in situ as a heptagon-containing C 68 Cl 6 (hepta-C 68 Cl 6 ). Carbon arc production and purification C 68 Cl 6 was produced in a Krätschmer–Huffman reactor of a graphite arc-discharge under 0.0395 atm CCl 4 and 0.1974 atm helium [29] , [31] . After separation and purification by multistage high performance liquid chromatography (HPLC), 1.6 mg of the C 68 Cl 6 of 99% purity was obtained from 150 g soot products of the CCl 4 -involving graphite arc-discharge (Methods; Supplementary Figs S1–S3 ). Crystallographic structure Single, black crystals suitable for X-ray diffraction were grown by solvent evaporation of a mixed solution of carbon disulfide and chloroform (2:1 in volume) of C 68 Cl 6 , ( Supplementary Figs S4 and S5 ; Supplementary Tables S1–S6 and Supplementary Methods ). 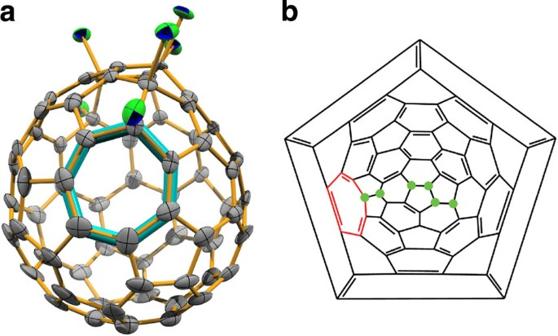Figure 1: Structure of C68Cl6molecule. ORTEP structure (a) and Schlegel diagram (b) of C68Cl6(ORTEP=Oak ridge thermal ellipsoid plot). The molecular structure of C 68 Cl 6 revealed by X-ray crystallography is shown in Figure 1 . It has 22 hexagons, 13 pentagons and 1 heptagon on the surface of the molecular cage. Of these, four pentagons are contiguous to form two pairs of doubly fused pentagons, in which the carbon atoms at the fusion are bonded to chlorine to relieve the unfavourable local strain. As well as the four chlorine atoms associated with these pentagon fusions, two further chlorines are bonded, one at each of two pentagon–hexagon–hexagon vertexes. The resultant sp 2 -hybridized 62-atom open-cage cluster is in good accord with the so-called Local aromaticity principle [32] . Figure 1: Structure of C 68 Cl 6 molecule. ORTEP structure ( a ) and Schlegel diagram ( b ) of C 68 Cl 6 (ORTEP=Oak ridge thermal ellipsoid plot). Full size image Mass spectrometric analysis The molecular composition of C 68 Cl 6 is confirmed by mass spectrometry (MS) ( Supplementary Fig. S3 ). Multistage mass spectrometric experiments show progressive dechlorination of C 68 Cl 6 and the eventual formation of bare C 68 , with the implication that heptafullerene[68] itself has a finite lifetime in the gas phase ( Fig. 2 ). 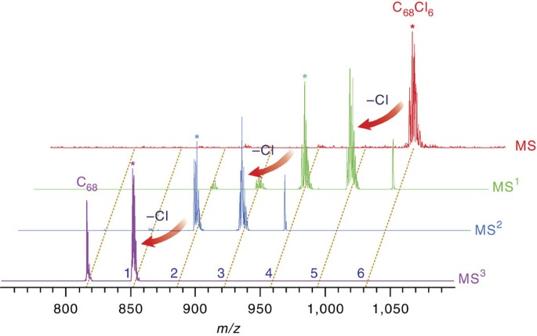Figure 2: Multistage mass spectrometry. (MSn,n=1–3). Progressive dechlorination produces C68Clm(m=0–6) (m is indicated in blue). The species picked for next stage of fragmentation, by collision with helium buffer gas in ion trap, is marked by an asterisk.m/z, mass to charge ratio. Figure 2: Multistage mass spectrometry. (MS n , n =1–3). Progressive dechlorination produces C 68 Cl m (m=0–6) (m is indicated in blue). The species picked for next stage of fragmentation, by collision with helium buffer gas in ion trap, is marked by an asterisk. m/z , mass to charge ratio. Full size image 13 C-Labelling experiments To establish that the retrieved C 68 species indeed grows together with other fullerenes in the CCl 4 -involving graphite arc-discharge conditions, a series of 13 C-labelled experiments were conducted in a glass chamber (inner diameter (I.D.) 194 mm) with reactants (graphite and CCl 4 ) having different 13 C contents: (A) Exp. A with normal graphite and CCl 4 (about 1.1 atm % 13 C); (B) Exp. B with 1.1 atm % 13 C graphite and 99 atm % 13 CCl 4 ; (C) Exp. C with 21.8 atm % 13 C-rich graphite and 1.1 atm % 13 CCl 4 . The products were analysed by HPLC–MS technology to record the mass spectra for individual components ( Supplementary Figs S6–S11 ). A total of 13 chlorinated polycyclic aromatic hydrocarbons (chloro-PAHs), 6 bare fullerenes, and 7 chlorofullerenes were detected in the crude products of the 13 C-labelled experiments ( Supplementary Figs S6–S11 ; Supplementary Table S7 ). Note that more species were detected when crude products were preliminarily concentrated by HPLC). 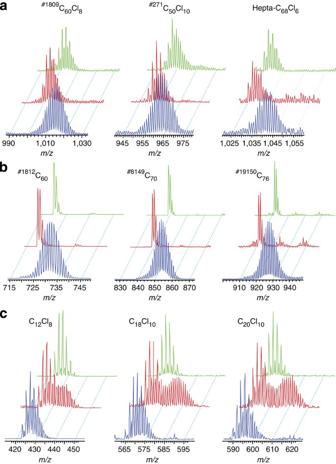Figure 3: Mass spectra of representative products from the13C-labelled experiments. The products are exemplified by (a) chlorofullerenes (#1809C60Cl8,#271C50Cl10and hepta-C68Cl6), (b) fullerenes (#1812C60,#8149C70and#19150C76) and (c) chloro-PAHs [C12Cl8, C18Cl10(2) and C20Cl10(1)]. Spectra are coloured green, red and blue for Expts. (A), (B) and (C), respectively.m/z, mass to charge ratio. Typical mass spectra of some selected products are shown in Figure 3 , including smaller chloro-PAHs (C 12 Cl 8 , C 18 Cl 10 (isomer 2) and C 20 Cl 10 (isomer 1)), typical fullerenes ( #1812 C 60 , #8149 C 70 and #19150 C 76 ), and chlorofullerenes ( #1809 C 60 Cl 8 , #271 C 50 Cl 10 and hepta-C 68 Cl 6 ). Note that the nomenclature specified by the Fowler–Manolopoulos spiral algorithm [33] has been used to distinguish classical non-heptagonal isomers. The mass spectrum of each product clearly shows the featured mass-to-charge ( m/z ) pattern ( Fig. 3 ; Supplementary Figs S6–S11 ). The m/z pattern can be clearly defined by the isotopic 12 C/ 13 C content of the corresponding cluster ( Supplementary Methods for details) and thus reflects the footprint of the parental carbon sources involved. Table 1 lists the estimated 13 C percentage of the selected carbon clusters according to the corresponding mass spectra recorded. Figure 3: Mass spectra of representative products from the 13 C-labelled experiments. The products are exemplified by ( a ) chlorofullerenes ( #1809 C 60 Cl 8 , #271 C 50 Cl 10 and hepta-C 68 Cl 6 ), ( b ) fullerenes ( #1812 C 60 , #8149 C 70 and #19150 C 76 ) and ( c ) chloro-PAHs [C 12 Cl 8 , C 18 Cl 10 (2) and C 20 Cl 10 (1)]. Spectra are coloured green, red and blue for Expts. (A), (B) and (C), respectively. m/z , mass to charge ratio. Full size image Table 1 The 13 C percentage estimated from mass spectra of selected carbon clusters produced in 13 C-labelled experiments. Full size table A classical cage-closed all-carbon structure (fullerene or carbon nanotube) typically contains a number of hexagons and exactly 12 pentagons. However, because of the incorporation of a heptagon, the number of pentagons in the present C 68 is increased to 13. Two pairs of them are adjacent, in violation of the isolated pentagon rule [22] , rendering the bare C 68 highly reactive and elusive. As a result of passivization by six chlorine atoms for the most reactive carbon atoms at the pentagon fusions and the aromaticity-unsatisfied sites, the elusive C 68 has been stabilized as chlorofullerene C 68 Cl 6 . The most prominent feature in the captured C 68 is the occurrence of a heptagon, which represents a new type of building unit for constructing cage-closed all-carbon architectures. In contrast to previously reported non-heptagonal fullerenes, heptafullerene[68] contains a heptagon having about 10% more space than a hexagon, and this presumably delivers easier pass through of foreign atoms, such as helium or nitrogen, to produce endofullerenes for potential technical applications. Indeed, first-principle density functional theory (DFT) calculations ( Supplementary Fig. S12 ; Supplementary Table S10 and Supplementary Methods ) predict that the activation energy for a helium atom penetrating into a fullerene cage decreases dramatically from 225.1 kcal mol −1 for I h -C 60 to 128.4 kcal mol −1 for hepta-C 68 Cl 6 . This easier penetration of helium into hepta-C 68 Cl 6 is also supported by mass spectrometric evidence ( Supplementary Fig. S13 ). The heptagon is surrounded by four pentagons and three hexagons. One of the carbon atoms in the heptagon is shared by two adjacent pentagons and subsequently transformed from sp 2 - to sp 3 -hybridization to release the strain of the doubly fused pentagons. Of interest is the decreased π-orbital axis vector (POAV) angle [34] of 6.0–10.4° (average 8.2°) at the fusions of the remaining two pairs of sp 2 -hybridized pentagon–heptagon junctions ( Fig. 1b ). These POAV angles are even smaller than those in the stable buckminsterfullerene I h -C 60 (11.64°), rendering heptafullerene[68] a heptagon-related planarity. Such kinds of decreased POAV angle have also been seen in the recently reported C 84 Cl 32 molecule, in which the POAV angles at the carbon atoms of the heptagon are in the range of 3.2–5.8° (average 5.2°) [28] . As the heptagon-related planarity facilitates strain relief in a curved surface of a cage, the existence of a heptagon may be expected to bring extra stabilization for the carbon cage involved. However, DFT calculations reveal substantial accommodation of the highest occupied molecular orbital electron densities around the cycloheptatriene-like ring of hepta-C 68 Cl 6 ( Supplementary Fig. S14 ; Supplementary Table S11 and Supplementary Methods ), implying a readiness for electrophilic additions at the heptagon area. DFT calculations also suggest that the C–Cl bond pertaining to the cycloheptatriene-like ring of hepta-C 68 Cl 6 is subject to nucleophilic substitution by taking advantage of local aromaticity of the 6-electron π-conjugated C 7 + tropylium-like ring in the corresponding hepta-C 68 Cl 5 + intermediate ( Supplementary Fig. S15 ; Supplementary Table S12 and Supplementary Methods ). Thus, the cycloheptatriene-like ring of hepta-C 68 Cl 6 is a double-edged sword, conveying unique reactivity to this heptagon-incorporating fullerene derivative, making it subject to both electrophilic addition and nucleophilic substitution. Theoretical studies predict that the hepta-C 68 has an energy comparable to that of the most stable isomers of classical C 68 that lack a heptagon. At room temperature, the hepta-C 68 is the third most stable of the C 68 isomers, with an energy ~2.5 kcal mol −1 higher than the most stable one. At a temperature above 2,100 K, however, the heptagon-incorporating C 68 becomes the most abundant species as entropic factors have a decisive role in their relative Gibbs free energies and relative concentrations/abundances ( Supplementary Tables S8 and S9 ). In agreement with this prediction about the temperature-dependent stability, several theoretical studies have suggested the prevalence of heptagons in the world of the cage-closed all-carbon allotropes [11] , [12] , [13] , [14] , [15] , [16] , [17] , [18] , [19] , [20] , [21] , [23] , [24] , [25] , [26] , [35] , [36] . Experimental corroboration of such a prevalence of heptagons heavily depends on the in situ capture of heptafullerene in the carbon clustering venue for the growth of the whole family of fullerenes. However, the previously reported heptafullerene derivatives (hepta-C 58 F 18 and hepta-C 84 Cl 32 ) were synthesized by an off-line top-down method through chemical detachment of a C 2 unit from a stable fullerene (C 60 or C 86 ) [27] , [28] . This top-down approach is similar to the so-called open-cage method in which the hexagons/pentagons of fullerene cages (typically C 60 ) are modified to give so-called open-cage fullerenes containing rings with twelve-, sixteen-, or eighteen-membered-rings and beyond [37] , [38] , [39] . By fluorination of C 60 at 550 °C, therefore, it is not surprising that two carbon atoms at a hexagon–pentagon fusion of C 60 have been removed to form stable derivatives of heptafullerene[58], C 58 F 18 or C 58 F 17 CF 3 (ref. 27 ). Very recently, the chlorinated heptafullerene[84] C 84 Cl 32 has also been synthesized from C 86 by chlorination at 250 °C (ref. 28 ). These cases, however, are inappropriate for establishing the survival of bare heptafullerenes in a bottom-up clustering process during growth of the whole fullerene family. In contrast, the present heptafullerene[68] molecule was captured in situ and directly isolated from the pristine products of a carbon arc, which is a typical venue for bottom-up growth of carbon allotropes such as fullerenes [29] , carbon nanotubes [2] and graphenes [30] . Powerful evidence to establish the bottom-up process comes from the 13 C-labelled Exp. C: the reactant of 21.8 atm % 13 C-rich graphite is an inhomogeneous mixture with a 90 atm % 13 C-rich carbon powder filled into a hollow graphite rod with regular 1.1 atm % 13 C content (Methods), but the produced hepta-C 68 Cl 6 and other fullerene species (for example, #1812 C 60 , #8149 C 70 , #19150 C 76 , #1809 C 60 Cl 8 , and #271 C 50 Cl 10 ) show an almost homogeneous 13 C percentage of 20.4 atm % (rather than the separated 1.1 or 90 atm % value) in the corresponding mass spectra ( Fig. 3 ; Supplementary Figs S9 and S10 ). This evidence, in accordance with previous literature [40] , [41] , [42] , clearly confirms that fullerenes grow from atomization of a carbon or small carbon clusters such as C 2 derived from graphite in the carbon arc process. Moreover, our 13 C-labelled experiments also ascertain that the bare heptafullerene[68] grows together with other fullerenes in the arc zone at high temperature and subsequently is captured by chlorine atoms produced from CCl 4 in the carbon arc conditions. In the present CCl 4 -involving graphite arc-discharge conditions, there are two carbon sources for the growth of carbon clusters, that is, the reactive carbon species from graphite (C-source I) and CCl 4 (C-source II). The former C-source I has a gradual density distribution with enhanced concentration at the arc zone but decreased beyond, whereas the latter CCl 4 source II is assumed to disperse in association with temperature distribution in the reaction chamber. The density of C-source I (or II) versus the distance from the arc centre (that is, the radius) in the reactor can be simulated based on mass conservation equation ( Supplementary Figs S16–S20 ; Supplementary Tables S13 , S14 and Supplementary Methods ). Accordingly, the carbon clusters produced at a certain region in the reactor can be quantified to grow from a mixture of carbon sources with an exclusive proportion of C-source I versus C-source II. In the present 13 C-labelled experiments, we conducted the syntheses of carbon clusters in a glass chamber (I.D. 194 mm) starting with the graphite and CCl 4 having different 12 C/ 13 C ratios, that is, Exp. A with normal graphite and CCl 4 (1.1 atm % 13 C), Exp. B with 1.1 atm % 13 C graphite and 99 atm % 13 CCl 4 , and Exp. C with 21.8 atm % 13 C-rich graphite and 1.1 atm % 13 CCl 4 . The products formed at a certain region inside the reactor would deliver an exclusive 12 C/ 13 C isotopic ratio that can be determined from the isotopic pattern recorded in the corresponding mass spectra (for example, Fig. 3 ). For example, the mass spectrum of hepta-C 68 Cl 6 itself shows the isotopic percentage of 13 C being ~1.6% 13 C in Exp. B and ~20.4% 13 C in Exp. C. Sequentially, the region for the growth of the carbon cluster product can be located simply according to the relationship of the 13 C isotopic percentage of products/reactants versus the location in the reactor for Exp. B or C ( Supplementary Figs S6–11, S16–20 ; Supplementary Tables S7, S13, S14 and Supplementary Methods ). 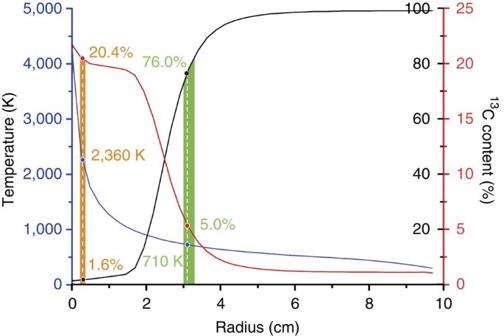Figure 4: Simulated curves of temperature and13C content. Simulated temperature (blue line) and13C content of carbon sources (black for Exp. B, red for Exp. C) versus distance from the arc centre (radiusr) for a reaction period of 600 s. Fullerenes with13C content of 1.6±0.1% in Exp. B and 20.4±0.1% in Exp. C are produced in an area ofr~2–3 mm at ~2,000–2,500 K (orange background) while a fraction of chloro-PAHs with13C content of 76.0±0.9 % in Exp. B and 5.0±0.4% in Exp. C are produced in an area ofr=~30–33 mm at ~700–730 K (green background). Figure 4 shows the simulated curves of 13 C content of reactive carbon sources (C-source I plus II) versus the distance from the arc centre in the reactor for Expts B and C (detailed calculations regarding mass conservation equation are described in Supplementary Methods ). According to the simulated curves and the estimated 13 C content in the hepta-C 68 Cl 6 produced from the 13 C-labelled experiments (Expts B and C), it can be concluded that the carbon framework of hepta-C 68 Cl 6 grows in the arc zone about 2–3 mm from the arc centre. Interestingly, as shown in the corresponding mass spectra ( Fig. 3 ; Supplementary Figs S6, S7, S9 and S10 ), isotopic percentages of 13 C in other representative fullerene species (for example, #1812 C 60 , #8149 C 70 , #19150 C 76 , #1809 C 60 Cl 8 , and #271 C 50 Cl 10 ) are approximately the same as those of hepta-C 68 Cl 6 itself, that is, ~1.1% 13 C in Exp. A, ~1.6% 13 C in Exp. B, and ~20.4% 13 C in Exp. C, implying that the heptafullerene[68] grows together with the other fullerenes in the same zone. Conformity of the reaction area with the experimentally obtained 13 C contents of fullerenes in both Exp. B and Exp. C validates the model of the mass conservation equation. Although the precision remains to be established, the proposed reaction zone might be informative for improving the yields of fullerenes in the carbon arc. As an example, we designed a synthetic experiment using a hollow anode (I.D. 4 mm) to replace a solid anode under otherwise identical arc-discharge conditions. Very interestingly, the yields of fullerene species such as #1812 C 60 , #8149 C 70 and #1809 C 60 Cl 8 were improved twofold ( Supplementary Fig. S21 and Supplementary Methods ), probably due to increase of the reaction venue at ~2 mm from the arc centre. Figure 4: Simulated curves of temperature and 13 C content. Simulated temperature (blue line) and 13 C content of carbon sources (black for Exp. B, red for Exp. C) versus distance from the arc centre (radius r ) for a reaction period of 600 s. Fullerenes with 13 C content of 1.6±0.1% in Exp. B and 20.4±0.1% in Exp. C are produced in an area of r ~2–3 mm at ~2,000–2,500 K (orange background) while a fraction of chloro-PAHs with 13 C content of 76.0±0.9 % in Exp. B and 5.0±0.4% in Exp. C are produced in an area of r =~30–33 mm at ~700–730 K (green background). Full size image The temperature for fullerene growth in a carbon arc is still uncertain. At the centre of the arc zone, the temperature could be higher than 4,000 K during the carbon-clustering process [43] . Beyond the arc zone, the temperature decreases rapidly. The relationship of temperature with the distance from the arc centre can also be simulated by an energy-conservation equation. The simulated temperature curve has been calibrated for good fit to the experimental data at sites of 34, 43 and 52 mm from the arc centre for a reaction time of 300 s ( Supplementary Figs S17 and S18 ). Because fullerenes grow at a region ~2 to 3 mm from the arc centre, the temperature region for fullerene growth can be estimated to be about 2,000–2,500 K from the simulated temperature curve ( Fig. 4 ). This estimate is in line with the above DFT prediction that hepta-C 68 is the most abundant isomer at a temperature higher than 2,100 K ( Supplementary Tables S8 and S9 ). It appears that at such a high temperature, Cl–C bonds can not survive and are likely irrelevant to the formation of pristine fullerenes. However, a drastic difference was observed in the mass spectra of smaller chlorinated carbon clusters, such as C 12 Cl 8 , C 14 Cl 8 (1, 2), C 16 Cl 10 (1–3), C 18 Cl 10 (1, 2) and C 20 Cl 10 (1–3) ( Fig. 3 and Table 1 , as well as Supplementary Figs S8, S11 and Supplementary Table S7 ). These smaller carbon clusters should have open structures similar to PAHs, because a carbon cluster of less than twenty carbon atoms is too small to give a cage structure. The Exp. B data exemplify that the corresponding mass spectra of these chloro-PAHs (red mass spectra in Fig. 3 ; Supplementary Fig. S8 ), very different from those of fullerenes ( Supplementary Figs S6 and S7 ), are a combination of two sets of m/z signals assignable to 13 C abundance ratios of approximately ~1.6 and ~76.0 atm % 13 C-rich species. Scrutiny of the mass spectra of Exp. C distinguishes two kinds of 13 C percentage (average ~5.0 and ~20.4 atm %) for the chloro-PAHs also ( Supplementary Fig. S11 ). Accordingly, two kinds of smaller carbon cluster can be established as growing from different reactive sources: one is produced in the high-temperature zone together with fullerenes and the other is formed in a chlorine-involving process in the region about 30–33 mm from the arc centre at ~700–730 K ( Fig. 4 ). The latter result is in accord with the fact that the smaller chlorinated PAHs can be produced from CCl 4 under pyrolysis conditions at around 600–1,000 K (refs 44 , 45 ), and, therefore, differentiates it from the formation mechanism of fullerene species. Such a formation difference between fullerenes and chloro-PAHs also corroborates that the parent heptafullerene[68] and other fullerenes grow in the high-temperature zone, independently of chlorine, and subsequently are captured/stabilized by chlorine on cooling outside the arc zone. The survival of heptafullerene in the carbon clustering process is thus clarified. On the basis of its crystallographic structure, the connectivity of hepta-C 68 also supports a hitherto unidentified mechanism for fullerene growth, namely the Heptagon road, in which the insertion of a C 2 cluster and the generation of heptafullerene have been suggested [46] . In the same carbon arc process, we have also been able to capture and isolate #4169 C 66 and #8149 C 70 (ref. 47 ). From a structural point of view, these two carbon clusters might be possible preceding/subsequent intermediates bridged by the heptafullerene[68]. 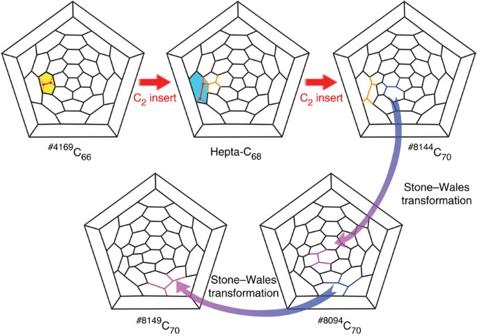Figure 5: Heptagon Road. Possible growth of fullerene from#4169C66to#8149C70through hepta-C68by the Heptagon Road and two Stone–Wales transformations. The scheme shown in Figure 5 suggests a possible route for the formation of #8149 C 70 by the Heptagon road involving C 2 -insertion growth from #4169 C 66 to #8144 C 70 , as well as two Stone–Wales transformations from #8144 C 70 to #8149 C 70 . It should be noted that this is just a possible implication simply inferred from the structures. Powerful evidence to elucidate the authentic mechanism is needed and further theoretical and experimental studies are now in hand. Figure 5: Heptagon Road. Possible growth of fullerene from #4169 C 66 to #8149 C 70 through hepta-C 68 by the Heptagon Road and two Stone–Wales transformations. Full size image In summary, heptafullerene[68] has been made and captured as chlorinated derivatives in a CCl 4 -involving graphite arc-discharge process. The 13 C-labelled synthetic experiments and mass/energy conservation equation simulations reveal that bare heptafullerene can grow in a bottom-up fashion in the arc zone at high temperature and survive in the gas phase during the carbon clustering process. This work, supported by X-ray crystallographic data and theoretical computations, fundamentally establishes that heptagon-incorporating fullerenes should not have been excluded in the classical fullerene family. It thus greatly increases the numbers of members of the fullerene family. The discovery of heptafullerene[68] may be expected to stimulate research activity in the field of all-carbon allotropes involving heptagons, for example: the synthesis of more heptagon-incorporating members in the family of carbon cages, understanding the formation mechanism(s) involving heptagons, and investigations of heptagon-dependent properties of carbon allotropes. Carbon arc production The carbonaceous soot containing fullerenes, chlorofullerenes, and smaller carbon clusters was produced under 0.1974 atm He and 0.0395 atm CCl 4 in a Krätschmer–Huffman arc-discharge reactor [29] , [31] , equipped with two graphite electrodes, a cathode cylinder block [40 mm (diameter)×60 mm], and an anode rod [8 mm diameter×300 mm]. An hourly production of about 3 g of soot was achieved for a power input of 33 V and 100 A. 13 C-labelled experiments The 13 C-labelled synthetic experiments were conducted in a glass chamber (I.D. 194 mm) starting with reactants (CCl 4 and graphite anode, diameter of 6 mm) having different 13 C contents. Exp. A was conducted with normal graphite and CCl 4 having the same 13 C percentage (about 1.1 atm %), Exp. B with 1.1 atm % 13 C graphite and 99 atm % 13 CCl 4 , and Exp. C with 21.8 atm % 13 C-rich graphite and 1.1 atm % 13 CCl 4 . The 13 C-rich graphite was prepared by filling 90 atm % 13 C-carbon powder into a regular 1.1 atm % 13 C hollow graphite rod. Isolation and identification Hepta-C 68 Cl 6 was extracted by toluene in an ultrasonic bath from the carbonaceous soot and purified by multistage HPLC process sequentially using a pyrenebutyric acid bonded silica column (I.D. 20×250 mm), a Cosmosil Buckyprep column (I.D. 10×250 mm), and a 5PPB column (I.D. 10×250 mm). All preparative HPLC were performed on a Shimadzu LC-6AD HPLC instrument at rt using toluene as eluent. HPLC–MS for the products from the 13 C-labelled synthetic experiments was analysed on a Discovery C18 column (I.D. 4.6×250 mm) of SUPELCO eluted by a methanol–ethanol–cyclohexane gradient. Mass spectra were recorded on a Bruker HCT mass instrument. Crystallographic data were collected on an Oxford CCD diffractometer ( Supplementary Methods ; Supplementary Data 1 ). How to cite this article: Tan Y-Z. et al . Carbon arc production of heptagon-containing fullerene[68]. Nat. Commun. 2:420 doi: 10.1038/ncomms1431 (2011).